Metal-induced rapid transformation of diamond into single and multilayer graphene on wafer scale The degradation of intrinsic properties of graphene during the transfer process constitutes a major challenge in graphene device fabrication, stimulating the need for direct growth of graphene on dielectric substrates. Previous attempts of metal-induced transformation of diamond and silicon carbide into graphene suffers from metal contamination and inability to scale graphene growth over large area. Here, we introduce a direct approach to transform polycrystalline diamond into high-quality graphene layers on wafer scale (4 inch in diameter) using a rapid thermal annealing process facilitated by a nickel, Ni thin film catalyst on top. We show that the process can be tuned to grow single or multilayer graphene with good electronic properties. Molecular dynamics simulations elucidate the mechanism of graphene growth on polycrystalline diamond. In addition, we demonstrate the lateral growth of free-standing graphene over micron-sized pre-fabricated holes, opening exciting opportunities for future graphene/diamond-based electronics. The exceptional electrical, thermal chemical, mechanical and optical properties of graphene are continuing to make strides in many fields [1] , [2] , [3] , [4] . The fabrication of devices [5] at the wafer scale for applications particularly related to the electrical and optical properties of graphene relies on a method that can produce large-area single-crystal graphene directly on dielectric substrates. The existing methods based on silicon carbide (SiC) [6] , [7] , [8] , [9] and hexagonal boron nitride (h-BN) [10] , [11] provide direct means of growing high-quality single-crystal graphene on these substrates. Another recently demonstrated method of wafer-scale growth of single-crystal graphene on germanium Ge (111) (refs 12 , 13 ) is also promising. The use of diamond as a substrate for supporting graphene is very appealing, as it offers several advantages and unique properties such as low trap density for charges, high energy for optical phonons, chemical inertness and high thermal conductivity [14] , [15] . In our previous studies on exfoliated graphene transferred onto ultrananocrystalline diamond (UNCD) thin films and single-crystal diamond [16] , we demonstrated that diamond offers an excellent platform for graphene by displaying a breakdown current density reaching up to 10 9 A cm −2 due to the excellent heat dissipation provided by the diamond under layer. It was demonstrated that replacing silicon dioxide (SiO 2 ) with diamond-like carbon allows one to improve radio-frequency characteristics on graphene transistors [17] . However, diamond-like carbon is an amorphous material with thermal conductivity K =0.2−3.5 Wm −1 K −1 at room temperature [4] , which is a very low value even when compared with SiO 2 . Synthetic diamond would be an ideal substrate for graphene devices in terms of its thermal properties, radio-frequency characteristics and compatibility with silicon complementary metal-oxide semiconductor technology. Although the technological benefits of having active material—graphene and substrate—diamond channels consisting of the same element (carbon) are tremendous, achieving this in practice remains a major synthesis and fabrication challenge. Transition metals, such as nickel [18] and iron [19] , have been used to demonstrate growth of multilayer and single-layer graphene on diamond (001) and (111) surfaces, respectively, by annealing them at high temperatures. However, in both cases, the resulting film still contains metals at the graphene–diamond interface, therefore not suitable for direct device fabrication. In addition, the size of graphene is limited by the size of the single-crystal diamond. In this letter, we report on a process for graphene synthesis, based on rapid thermal annealing of a UNCD film in the presence of a metal catalyst, such as Ni. A distinguishing feature of our process is the elimination of the need for any transfer process. More importantly, we also demonstrate interesting features of lateral growth of suspended graphene over micron-sized holes where graphene appears to be single domain as demonstrated later with selected area electron diffraction technique performed on the graphene transferred from various places onto transmission electron microscope (TEM) grid. This is very important for practical applications, where devices could be fabricated over suspended graphene. In addition, the graphene can be grown selectively just by patterning the deposition of metal at micron scale. Graphene on UNCD films and their properties The rapid thermal annealing process ( Fig. 1a ) presented here is capable of producing graphene on polycrystalline diamond sample and Raman spectroscopy analysis carried out at different locations clearly indicates graphene coverage all over the 4-inch diameter wafer ( Fig. 1b–g ). We choose UNCD as a substrate as it offers unique properties that no other diamond film provides due to its small grain size (2–5 nm) and high-volume fraction of grain boundaries. A 50-nm Nickel film was deposited on the UNCD surface by e-beam evaporation. As a result, during thermal annealing process ( Fig. 1a ), nickel diffuses rapidly through the UNCD grain boundaries as compared with through UNCD grains and sits at the bottom of the UNCD/Si interface. Due to the rapid diffusion of Ni during the temperature ramp, only a small amount of Ni is left over on the top in the form of islands (which also eventually diffuses in diamond), which act as nucleation centres for the graphene growth. The continuous supply of carbon from the UNCD underneath enables the rapid lateral growth of graphene at the wafer scale. The graphene films produced by this method were characterized using X-ray photoemission spectroscopy (XPS) demonstrating its high-quality nature through the clear carbon signature without any indication of the presence of nickel on the surface after the annealing process ( Fig. 2 ). Cross-section scanning electron microscopy (SEM) corroborates the complete nickel segregation to the bottom of the UNCD layer ( Supplementary Fig. 1 ). Also, detailed analysis of the carbon peak in the XPS high-resolution scan ( Fig. 2b ) demonstrates the presence of only sp 2 bonded carbon on the surface, hence indicating the high-purity nature of the obtained graphene, without any modification (such as oxidation). 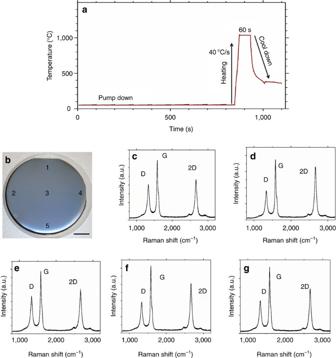Figure 1: Wafer-scale growth of graphene on diamond. (a) Recipe for the thermal annealing process shows rapid heating of the sample’s temperature up to 1,000 °C, keeping the system at high temperature for 60 s followed by rapid cooling down to room temperature. (b) A photograph of the 4-inch diameter wafer covered with graphene after the annealing process is shown and the Raman analysis of the sample at five random spots is presented. (c) Corresponds to spot 1, (d) to spot 2, (e) to spot 3, (f) to spot 4 and (g) to spot 5. Scale bar, 2 cm (b). Figure 1: Wafer-scale growth of graphene on diamond. ( a ) Recipe for the thermal annealing process shows rapid heating of the sample’s temperature up to 1,000 °C, keeping the system at high temperature for 60 s followed by rapid cooling down to room temperature. ( b ) A photograph of the 4-inch diameter wafer covered with graphene after the annealing process is shown and the Raman analysis of the sample at five random spots is presented. ( c ) Corresponds to spot 1, ( d ) to spot 2, ( e ) to spot 3, ( f ) to spot 4 and ( g ) to spot 5. Scale bar, 2 cm ( b ). 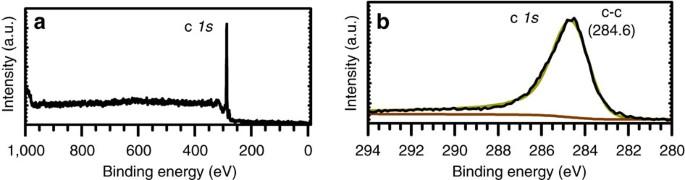Figure 2: XPS analysis of the graphene on diamond sample. (a) The full survey XPS scan of the sample demonstrates the presence of prominent carbon C1speak on the surface, indicating absence of residual nickel on the surface as well as no oxygen presence. (b) detailed carbon C1speak confirmssp2hybridization of graphene through presence of C–C bond peak highlighted in green. Black colour indicates the collected XPS data and brown highlights the background spectra. Full size image Figure 2: XPS analysis of the graphene on diamond sample. ( a ) The full survey XPS scan of the sample demonstrates the presence of prominent carbon C 1s peak on the surface, indicating absence of residual nickel on the surface as well as no oxygen presence. ( b ) detailed carbon C 1s peak confirms sp 2 hybridization of graphene through presence of C–C bond peak highlighted in green. Black colour indicates the collected XPS data and brown highlights the background spectra. Full size image Surface analysis of the produced wafer indicates growth of a continuous graphene film ( Supplementary Figs 2 and 3 ). The SEM ( Fig. 3a ) and atomic force microscopy (AFM) ( Fig. 3b ) images demonstrate the surface morphology of the as-grown film, displaying a smooth surface (root mean square roughness R q =0.8 nm) with only occasional folds of the graphene layer (areal density, defined as the area under the wrinkles divided by the total scanning area, is <0.5%). We believe that these folds as seen on the AFM image ( Fig. 3b ) may also contribute to the defect peak D (at ∼ 1,335 cm −1 ) in the Raman signature [20] ( Fig. 3c ) along with underlying UNCD. The presence of the folds could be attributed to uneven distribution of stress as a consequence of the fast annealing process. 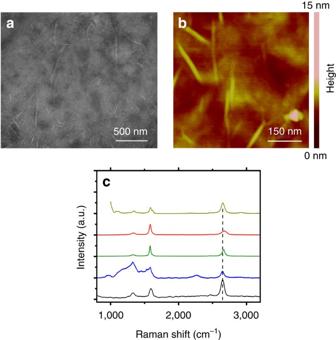Figure 3: Characterization of graphene on UNCD sample. (a) The SEM and (b) AFM images of grown graphene indicate the formation of the continuous uniform film with occasional folds occurring; (c) Raman signature of graphene films produced at different temperatures indicates the variation in the number of grown layers (green line highlighting single layer grown at 800 °C and red line highlighting multilayer grown at 1,000 °C). The Raman signature of graphene grown at 800 °C and then thermal-release tape transferred onto silicon dioxide substrate (dark yellow) confirms the single-layer thickness of graphene. The Raman spectra of single-layer graphene grown on copper (black line) and then transferred on the UNCD film (blue line) are provided for reference. Dashed line highlights the position of 2D peak. Figure 3: Characterization of graphene on UNCD sample. ( a ) The SEM and ( b ) AFM images of grown graphene indicate the formation of the continuous uniform film with occasional folds occurring; ( c ) Raman signature of graphene films produced at different temperatures indicates the variation in the number of grown layers (green line highlighting single layer grown at 800 °C and red line highlighting multilayer grown at 1,000 °C). The Raman signature of graphene grown at 800 °C and then thermal-release tape transferred onto silicon dioxide substrate (dark yellow) confirms the single-layer thickness of graphene. The Raman spectra of single-layer graphene grown on copper (black line) and then transferred on the UNCD film (blue line) are provided for reference. Dashed line highlights the position of 2D peak. Full size image To produce graphene films with different thicknesses, we varied the temperature of the process from 800 °C to up to 1,000 °C ( Fig. 3c ). It is important to note subtle differences in the Raman spectra of the single-layer graphene directly grown on UNCD versus single-layer graphene, grown initially on copper by chemical vapour deposition and subsequently transferred onto the UNCD surface. Due to substrate effects caused by the underlying UNCD film [15] , the Raman signature shows the presence of a defect peak D (at ∼ 1,335 cm −1 ) and low-intensity ratio second order defect peak of 2D (at ∼ 2,650 cm −1 ) to G (at ∼ 1,585 cm −1 ) bands I 2D / I G =0.6 in comparison with that of a single-layer graphene ( I 2D / I G =2) (refs 21 , 22 ), grown on copper foil ( Fig. 3c ). Moreover, significant blue shifts on both, G and 2D bands, as well as an increased 2D-band full-width half maximum are observed for these graphene films on UNCD. This effect may occur due to strong interfacial bonding between graphene and UNCD, which produces strain that manifests itself as the shift observed in the 2D bands. A similar effect has been observed for graphene grown on SiC substrates [23] . For annealing temperatures as low as 800 °C, the Raman signature indicates significantly reduced number of graphene layers [24] , [25] , whereas for annealing at higher temperatures (1,000 °C), the resulting graphene films are multilayered and display a smoother morphology (root mean square roughness decreases from 1.43 nm for single-layer graphene at 800 °C down to 0.8 nm for multilayer graphene at 1,000 °C). Therefore, the thickness of the graphene film can be tuned by varying the annealing temperature. However, it is important to mention that we managed to achieve either single or multilayer graphene only, due to constraints on our experimental setup, mainly involving the fast, precise control of temperature ramping. The quality of the graphene films grown on UNCD was also evaluated by measuring the sheet resistance using the four-point probe method. The sheet resistance of the obtained graphene/UNCD films varied from 0.09 Ω per square for thick (20–30 nm) graphene samples grown at 1,000 °C to 3.1 Ω per square for single-layer graphene grown at 800 °C. This is the lowest value of sheet resistance reported so far for multilayer, bilayer and doped free-standing single-layer graphene [26] , [27] , [28] , which we attribute to the high quality of the produced graphene. We have also fabricated graphene top-gate field-effect transistors. The current–voltage ( I–V ) characteristics of the top-gated devices were measured using a semiconductor parameter analyzer ( Fig. 4 ). The linearity of the source-drain current versus source-drain voltage ( I ds versus V ds ) curve ( Fig. 4a ) confirms the high-quality Ohmic contact. The V-shape of source-drain current as a function of the gate bias ( I ds – V g ) curve ( Fig. 4b ) is characteristic for graphene and indicates that the charge carrier type can be switched from electrons to holes by tuning the gate bias. The calculated electron mobility at room temperature ∼ 2,000 cm 2 V −1 s −1 with carrier density of 3.5 × 10 12 cm −2 indicates suitability for radio-frequency applications. 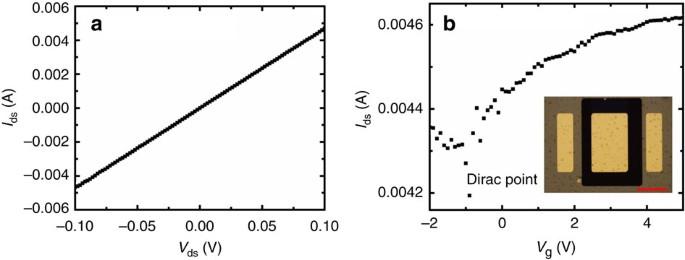Figure 4: Top gate field-effect transistor fabricated on graphene on diamond. (a) Two terminal current–voltage characteristicsIdsversusVdsat zero gate bias. (b) Three-terminal measurement source-drain current versus top-gate bias. Drain voltage is fixed at 0.1 V. Scale bar, 100 μm. The dark part is a dielectric layer of HfO2with the size of 200 μm by 300 μm. The gate electrode is 200 μm in width and 120 μm in length. The source and drain electrodes are 200 μm in width and 50 μm in length. Figure 4: Top gate field-effect transistor fabricated on graphene on diamond. ( a ) Two terminal current–voltage characteristics I ds versus V ds at zero gate bias. ( b ) Three-terminal measurement source-drain current versus top-gate bias. Drain voltage is fixed at 0.1 V. Scale bar, 100 μm. The dark part is a dielectric layer of HfO 2 with the size of 200 μm by 300 μm. The gate electrode is 200 μm in width and 120 μm in length. The source and drain electrodes are 200 μm in width and 50 μm in length. Full size image In addition to producing high-quality planar sheets of graphene directly onto UNCD surfaces, free-standing graphene films were successfully grown over holes made in diamond ( Fig. 5 and Supplementary Fig. 4 ). 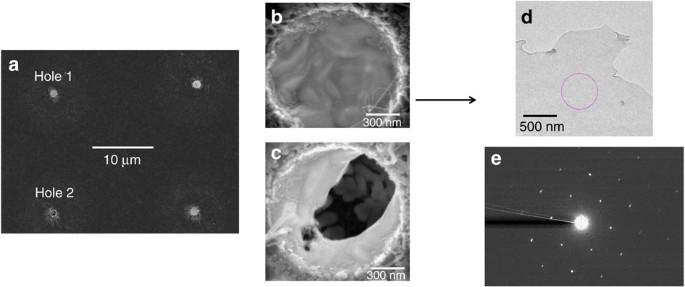Figure 5: Lateral growth of single domain free-standing graphene on diamond. (a) Successful growth of graphene on four holes is presented. (b) Full coverage of hole 1 is demonstrated. (c) Graphene partially grown on the hole 2 confirms free-standing nature. (d) TEM image confirms a single-domain graphene growth with (e) selected area electron diffraction (SAED) pattern indicating diffraction of single-domain graphene film. The circle indhighlights the area where SAED pattern was recorded. Figure 5a demonstrates that annealing of the Ni/UNCD sample resulted in three holes being completely covered with graphene while one remaining hole was only partially covered. Lateral growth of graphite layers under a thermal gradient was theoretically predicted by Ye et al. [29] . Here, however, we present an experimental evidence of such successful lateral graphene growth. We should emphasize, that the successful growth of free-standing graphene is limited by the size of the hole and the presence of nickel in close proximity. Also, we demonstrate that just by patterning the nickel film, a selective growth of graphene can be obtained at predefined locations on diamond ( Supplementary Fig. 5 ). X-ray diffraction analysis ( Supplementary Fig. 6 ) showed predominantly Ni (111) crystal plane orientation of the evaporated nickel films on UNCD. Figure 5: Lateral growth of single domain free-standing graphene on diamond. ( a ) Successful growth of graphene on four holes is presented. ( b ) Full coverage of hole 1 is demonstrated. ( c ) Graphene partially grown on the hole 2 confirms free-standing nature. ( d ) TEM image confirms a single-domain graphene growth with ( e ) selected area electron diffraction (SAED) pattern indicating diffraction of single-domain graphene film. The circle in d highlights the area where SAED pattern was recorded. Full size image To determine the quality of the free-standing graphene films, samples were transferred to TEM grid. The selected area electron diffraction pattern demonstrates the single-domain graphene layer ( Fig. 5d,e ). Detailed Raman study of the graphene on the hole indicates lowering the intensity of the defect peak D (at ∼ 1,335 cm −1 ) and increasing the intensity of 2D (at ∼ 2,650 cm −1 ) peak due to the reduced coupling with the UNCD underneath, though the signature does not correspond yet to the single-layer graphene due to shallow shape and small size (500 nm) of the hole ( Fig. 6 ) as compared with the Raman spot size (1.2 μm). In addition, to confirm the single-layer nature of the graphene, we have been able to transfer some part of the graphene on a SiO 2 -coated Si substrate (although with some difficulty) using a thermal release tape and the corresponding Raman signature confirms single-layer signature of graphene ( Supplementary Fig. 2 ). 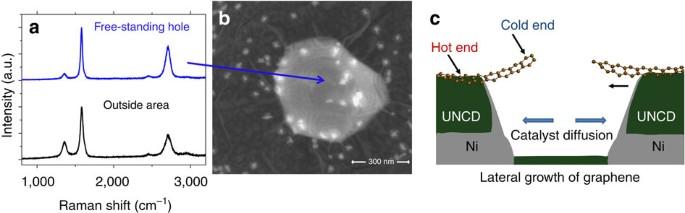Figure 6: Growth mechanism of free-standing graphene. (a) Changes in the intensities of D and 2D peaks for Raman signature of the graphene on the hole (fromID/IG=0.3 andI2D/IG=0.4 outside the hole toID/IG=0.1 andI2D/IG=0.6) indicate growth of the free-standing graphene. (b) The Raman signature of graphene grown directly on UNCD (outside area) is provided for the reference. (c) The schematic of mechanism of free-standing graphene growth is presented. Figure 6: Growth mechanism of free-standing graphene. ( a ) Changes in the intensities of D and 2D peaks for Raman signature of the graphene on the hole (from I D / I G =0.3 and I 2D / I G =0.4 outside the hole to I D / I G =0.1 and I 2D / I G =0.6) indicate growth of the free-standing graphene. ( b ) The Raman signature of graphene grown directly on UNCD (outside area) is provided for the reference. ( c ) The schematic of mechanism of free-standing graphene growth is presented. Full size image Atomic-scale mechanism of the graphene formation on diamond To gain insights into the atomic-scale mechanisms underlying the formation of graphene on diamond on rapid annealing Ni/polycrystalline UNCD films, we turn to reactive molecular dynamic (MD) simulations ( Supplementary Note 1 ). Previous studies have successfully employed MD simulations to investigate the atomic-scale processes governing the nucleation and subsequent growth of graphene and carbon nanotubes on transition metal surfaces; [30] , [31] , [32] a comprehensive review on this topic has been recently published by Elliot and co-workers [33] . In those studies, the carbon atoms were deposited on transition metal surfaces (usually Ni) at various rates and were assumed to arise by decomposition of hydrocarbons for example, in chemical vapour deposition (CVD). The Ni/UNCD films used in the present study, however, pose hitherto unanswered questions related to interaction between Ni films and UNCD grain boundaries, as well as associated atomic transport phenomena; such an understanding is crucial to gain precise control over synthesis of monolayer/few-layer graphene from Ni/UNCD films. To investigate these phenomena, we performed two sets of simulations. First, we anneal Ni (111) slab placed on top of a typical grain boundary (GB), namely, Σ13 twist (100) in UNCD at various temperatures 1,200–1,600 K ( Supplementary Fig. 7 ). Here we focus on the counter-diffusion of carbon (C) and Ni at the Ni/UNCD interface, and the evolution of the structure at the interface. The concurrence of these events eventually leads to the nucleation of graphene islands on the free surface. In the second set, we investigate the diffusion of C atoms on free Ni surface, which assists rapid lateral growth of the formed graphene nuclei. For this set, we deposited several C atoms at random locations on Ni (111) and Ni (001) surfaces ensuring identical C coverage. These two sets of simulations provide a holistic picture of the atomic-scale events leading to the nucleation and growth of graphene on annealing of Ni/UNCD films ( Fig. 7 ). 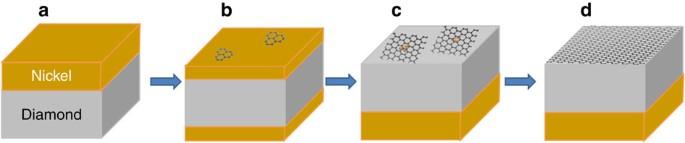Figure 7: Schematic of the Ni (111)-facilitated graphene growth. Subsequent growth procedure of graphene starting from initial Ni/UNCD (a) configuration with following nucleation (b) and increase in domain size (c) of graphene up to full coverage (d). Figure 7: Schematic of the Ni (111)-facilitated graphene growth. Subsequent growth procedure of graphene starting from initial Ni/UNCD ( a ) configuration with following nucleation ( b ) and increase in domain size ( c ) of graphene up to full coverage ( d ). Full size image Our first set of simulations on Ni (111)/UNCD interface capture the sequence of atomic scale events leading to graphene nucleation on Ni (111). Initially, Ni atoms penetrate into the UNCD GB, which, in turn, introduces structural disorder near the GB, and eventually leads to rapid amorphization of UNCD ( Supplementary Movie 1 ). Concurrently, the C atoms from the amorphous region dissolve into the Ni thin film; this dissolution continues until the Ni film gets saturated with C atoms. At the annealing temperatures employed in this study (1,200–1,800 K), the solubility of C in Ni is known to be ∼ 1–2% (ref. 34 ), which is well described by the reactive force field (ReaxFF) used in this study ( Supplementary Note 2 ) [35] . Beyond the solubility limit, the C atoms proximal to the free Ni surface precipitate out, and eventually result in graphene-like C-rings ( Fig. 8 ). Once these rings (nuclei) form, they grow rapidly in the lateral dimensions through diffusion of C atoms over the free Ni surface ( Fig. 9 ). These events involving C super-saturation of Ni films, and precipitation of C on Ni surfaces are analogous to earlier MD reports on formation of graphene on transition metal surfaces during CVD synthesis [16] , [36] , [37] , [38] , [39] , [40] , [41] . We note that the rate of nucleation of these graphene-like C rings is governed mainly by the concurrent counter-diffusion of Ni and C, and the consequent amorphization of the Ni/UNCD interface. 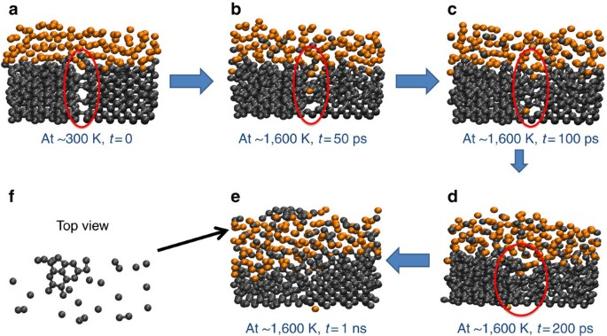Figure 8: Carbon diffusion through the diamond grain boundaries mechanism. Carbon diffusion through the nickel film and eventual segregation of nickel through diamond grain boundaries is highlighted through MD simulations: (a) initial configuration shows nickel film on two diamond grains, (b) heating up to 1,600 K for 50 ps indicates segregation of nickel atoms through the grain boundary, (c) at 100 ps one nickel atom diffuses all the way down to the bottom of diamond, (d) more nickel atoms segregate at 200 ps and top layer of diamond starts to graphitize, (e) indicates the formation of graphitic layer on top of nickel, and (f) top view depicts the formation of graphene rings. Carbon atoms are represented by dark grey colour, while nickel atoms by dark orange colour. Red oval highlights the grain boundary. Figure 8: Carbon diffusion through the diamond grain boundaries mechanism. Carbon diffusion through the nickel film and eventual segregation of nickel through diamond grain boundaries is highlighted through MD simulations: ( a ) initial configuration shows nickel film on two diamond grains, ( b ) heating up to 1,600 K for 50 ps indicates segregation of nickel atoms through the grain boundary, ( c ) at 100 ps one nickel atom diffuses all the way down to the bottom of diamond, ( d ) more nickel atoms segregate at 200 ps and top layer of diamond starts to graphitize, ( e ) indicates the formation of graphitic layer on top of nickel, and ( f ) top view depicts the formation of graphene rings. Carbon atoms are represented by dark grey colour, while nickel atoms by dark orange colour. Red oval highlights the grain boundary. 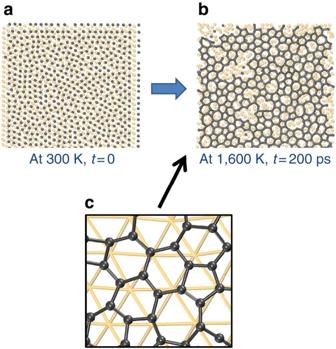Figure 9: Growth of graphene film on Ni (111) surface. Growth of uniform graphene film on Ni (111) surface is highlighted. (a) Initially, amorphous carbon is placed on Ni (111) film. (b) After heating up to 1,600 K for 200 ps formation of ordered graphene rings on the nickel surface is observed with (c) high-magnification image indicating lattice configuration of graphene on nickel. Carbon atoms are represented by dark grey colour, while nickel atoms by pale orange colour. Full size image Figure 9: Growth of graphene film on Ni (111) surface. Growth of uniform graphene film on Ni (111) surface is highlighted. ( a ) Initially, amorphous carbon is placed on Ni (111) film. ( b ) After heating up to 1,600 K for 200 ps formation of ordered graphene rings on the nickel surface is observed with ( c ) high-magnification image indicating lattice configuration of graphene on nickel. Carbon atoms are represented by dark grey colour, while nickel atoms by pale orange colour. Full size image We ascertain that the presence of GBs in UNCD assists the nucleation of graphene on free Ni surfaces ( Supplementary Note 3 ). MD simulations using Ni(111) on single-crystal diamond ( Supplementary Fig. 8 ) conclusively showed that the kinetics of Ni dissolution into the UNCD is severely impaired in the absence of GB. This, in turn, restricts the amorphization of the UNCD within 1–2 layers of the Ni/UNCD interface within MD timescales ( ∼ 2 ns), and limits the C flux into Ni slab to a few atoms. Thus, in the absence of UNCD GB, the transport of C to the free Ni surface is negligible. Our MD simulations ( Supplementary Note 4 ) of surface diffusion of C atoms from random locations on Ni surfaces ( Fig. 9 ) indicate that the diffusion of C over a Ni surface occurs over timescales (in the order of tens of ps) that are much faster than those for nucleating graphene islands (in the order of ns). This result is valid irrespective of the crystallographic orientation of Ni surface. Such a distinct difference between the kinetics of nucleation and growth phases is ideal for forming single-domain graphene sheets. The growth kinetics of graphene is particularly favourable on the Ni (111) surface ( Supplementary Fig. 9 ) owing to low diffusion barrier for C on Ni (111) of 0.5 eV (ref. 42 ). In addition, the Ni atoms on (111) plane are arranged on a close-packed triangular lattice ( Fig. 9c ), which closely imitates the honeycomb structure of graphene. This commensurability between Ni (111) substrate and graphene enables the growth of graphene nuclei into large domains, which are mostly uniform and defect-free. Our simulations suggest that the diffusivity of C through the Ni film is much faster than the rate of depletion of Ni at the Ni–GB interface, thereby ensuring that the (111) preferred orientation of the free surface is preserved. On the Ni (111) surface, we observe another interesting behaviour exhibited by the C atoms. Initially, the C atoms diffuse rapidly on the Ni (111) surface and bind to neighbouring C atoms in the form of rings, which may either be graphitic (six-membered) or defective (non six-membered, for example, in Stone–Waals defects). Once a continuous largely planar network of the C atoms is formed, the re-arrangement of C atoms continues, which results in healing of defects (that is, conversion of defective rings into graphitic ones). This re-arrangement can be attributed to the template provided by the underlying Ni (111), and does not occur over Ni (001) ( Supplementary Fig. 9 ). Consequently, the monolayer graphene that forms on Ni (111) surface features the least number of defects, and covers nearly the entire substrate ( Fig. 9 ). We note that these results are robust; the effect of the Ni surface orientation on graphene growth is unaffected by the temperature schedule and the highest temperature achieved during the annealing. The kinetics of re-organization of C-atoms to reduce the defects, as expected, is slow at lower temperatures. These simulation results are in good qualitative agreement with experimental observations. Overall, the general picture that emerges from our experimental results and well-supported by simulations is that graphene nucleation and growth occurs on Ni (111) surface and is much faster than Ni diffusion into UNCD GBs, therefore graphene growth occurs first followed by complete diffusion of Ni into the UNCD bottom leaving intact a uniform graphene layer on top of the UNCD. In summary, we have demonstrated a process of growing high-quality wafer-scale graphene film directly onto an insulating substrate by rapid thermal annealing of diamond film in the presence of a metal catalyst. This is very promising as our process does not involve transferring of graphene over other substrate. The tuning of the graphene thickness is achieved through the variation of the annealing temperature such that, at lower temperatures (800 °C) the obtained graphene film consists of a single layer, while increasing the annealing temperature to up to 1,000 °C results in multilayer graphene. Reactive MD simulations elucidate an intriguing kinetically controlled mechanism of graphene nucleation and growth facilitated by Ni-induced amorphization of diamond. This fabrication scheme can be easily extended to form suspended graphene membranes directly on diamond. This opens up more avenues to exploit full advantages of intrinsic properties of suspended graphene. Thus, the graphene-on-diamond platform is promising for the development of high performance, energy-efficient nanoelectronic devices. Fabrication procedure UNCD film is grown by a microwave plasma-enhanced CVD (MPCVD) process using an Ar-rich/CH 4 chemistry (Ar (99%)/CH 4 (1%)) on silicon substrate [43] . The thickness of UNCD films varied from 200 nm up to 300 nm, measured with Spectroscopic Reflectometer SR 300. A 50-nm nickel film was deposited on the UNCD surface by e-beam evaporation using a Kurt J Lesker PVD250 e-beam evaporator with a base pressure of ∼ 10 −8 torr and a deposition rate of 5 Å s −1 , which, along with the low base pressure, provides high-purity nickel film (source: pellets 99.995% pure). The thickness of the nickel film was controlled by quartz crystal monitor pre-calibrated before the deposition process using a lithographic patterning, thus guaranteeing <1% thickness variation during the deposition. After this, the samples were processed in a rapid thermal annealing system (ramping speed 40° s −1 ) in a temperature range between 800 and 1,000 °C for 60 s while flowing 500 s.c.c.m. of the forming gas mixture (5% of H 2 and 95% of N 2 ). This procedure proved to be effective for growing uniform graphene layers on UNCD surfaces. Free-standing graphene The free-standing graphene samples were obtained using the specific procedure. Initially, SEM ion milling was used to make holes, 500 nm deep, on UNCD films and then 50 nm Ni film was evaporated. The holes had diameters varying from 300 nm up to 1 μm. Afterwards, to produce lateral growth of graphene over the holes, RTA annealing steps were performed following the same procedure as described for the plain UNCD sample. Characterization XPS analysis was performed by a home-built X-ray photoelectron spectrometer, which includes a hemispherical electron energy analyzer of 0.9 eV energy resolution and a non-monochromated Mg K-alpha soft X-ray source at 1,253 eV. Raman spectroscopy analysis has been performed by an Invia Confocal Raman Microscope using the red laser light (wavelength λ =633 nm) to confirm the formation of a graphene layer on the UNCD surface. The intensity and position of the characteristic G and 2D graphene peaks, as well as the full width at half maximum of the 2D peak in the Raman spectra show the variation in the number of graphene layers grown at different temperatures. The presence of defect peak D can be explained by graphene folds clearly seen in SEM and AFM images ( Fig. 3 ). SEM images were obtained using a FEI Nova 600 Nanolab dual-beam microscope with focused ion beam used for making the cross-section of the grown layers. To protect the sample, two platinum films are deposited on the surface before making the cross-section. Energy-dispersive X-ray spectroscopy analysis of the layers confirmed the position of nickel layer (as shown in Supplementary Fig. 1 ) before and after annealing, and carbon layer, confirming nickel segregation inside the UNCD and thus producing direct graphene deposition on the diamond surface. AFM measurements were performed to demonstrate the three-dimensional structure of the grown layers. For this purpose, the images were acquired by an AFM Veeco Microscope at ambient air conditions (relative humidity ∼ 30%) using a n -doped silicon tip in tapping mode. TEM studies were performed on two different types of samples: grown graphene layer and the cross-section of graphene grown on UNCD. In the first case, the sample was prepared by using thermal release tape to transfer the top layer on the TEM 300 mesh copper grid. In the second case, the sample was prepared using focused ion beam at the SEM instrument, when the sample was cut at the cross-section and then attached to the TEM lift-out grid using focused ion-beam milling. Observation of the single-domain graphene is performed using TEM JEOL JEM-2100F. X-ray diffraction analysis was performed with Bruker D2 Phaser Diffractometer to demonstrate the crystal orientation of the grown nickel films on UNCD wafer. Graphene on diamond-based transistors To test the electron mobility of the CVD-grown graphene on UNCD substrates, we fabricated a number of graphene top-gate field-effect transistors. The top-gate dielectric layer that consists of 20-nm-thick HfO 2 was grown by atomic layer deposition. The electron beam lithography technique was used to define the source, drain and gate electrodes. Ti/Au films with thickness of 10 nm/100 nm were deposited by electron beam evaporation to form the metal contact to the devices. The current–voltage ( I–V ) characteristics of the top-gated devices were measured using a semiconductor parameter analyzer. First, the source-drain current versus source-drain voltage was measured at zero gate bias with two terminal measurements. Second, for the source-drain current as a function of the gate bias curve, the source-drain voltage was kept at 0.1 V while the gate bias swept from −2 to 5 V. The Dirac point of the tested device is around −1 V. The carrier mobility of electrons and holes can be extracted using the Drude formula (equation (1)): where is the transconductance, is the gate capacitance per area, where the relative permittivity of HfO 2 is 25. L g and W are the length and width of the gate, respectively. The electron mobility at ∼ 2,000 cm 2 V −1 s −1 was obtained at −0.5 V gate bias. The carrier density was 3.5 × 10 12 cm −2 at this point. The maximum gate bias applied was +5 V and carrier density was ∼ 4.2 × 10 13 cm −2 . Molecular dynamic simulations We employed reactive MD simulations to investigate the atomic-scale events leading to the formation of graphene domains on the surface of diamond during thermal annealing of thin films comprising of Ni and polycrystalline UNCD. To explore the nucleation and growth of graphene in this complex system within timescales afforded by MD simulations, we performed two sets of simulations. First, we probe the atomic-scale events leading to the nucleation of graphene (few six-membered C rings) on the free surface on annealing a system consisting of Ni placed onto a UNCD bicrystal containing a typical twist GB. The methods used to generate the computational supercell are detailed in Supplementary Note 1 . The thermal annealing was performed at various temperatures in the range 1,200–1,600 K. The conclusions from all these simulations are identical, except as expected, the frequency of occurrence of these events decreases at lower temperatures. The events leading up to the nucleation, as detailed in the main manuscript, consist of penetration of Ni into UNCD GB causing disorder near the GB, propagation of this disorder leading to amorphization of UNCD, transport of C from amorphous region to the Ni film, supersaturation of Ni with carbon, and precipitation of C on the free surface, which forms carbon rings (assisted by commensurability of Ni (111) and graphene). In the second set, we study the fast kinetics of growth of graphene nucleus (that occurs over tens of ps). Here we deposit carbon atoms at random locations on the free surface of a Ni slab and monitor the formation of C rings on annealing at different temperatures. We have also studied the effect of crystallographic orientation of the Ni slab. Additional details on the simulations can be found in Supplementary Note 4 . Data availability The data that support the findings of this study are available from the corresponding author upon request. How to cite this article: Berman, D. et al. Metal-induced rapid transformation of diamond into single and multilayer graphene on wafer scale. Nat. Commun. 7:12099 doi: 10.1038/ncomms12099 (2016).